Experimental implementation of bit commitment in the noisy-storage model Fundamental primitives such as bit commitment and oblivious transfer serve as building blocks for many other two-party protocols. Hence, the secure implementation of such primitives is important in modern cryptography. Here we present a bit commitment protocol that is secure as long as the attacker’s quantum memory device is imperfect. The latter assumption is known as the noisy-storage model. We experimentally executed this protocol by performing measurements on polarization-entangled photon pairs. Our work includes a full security analysis, accounting for all experimental error rates and finite size effects. This demonstrates the feasibility of two-party protocols in this model using real-world quantum devices. Finally, we provide a general analysis of our bit commitment protocol for a range of experimental parameters. Traditionally, the main objective of cryptography has been to protect communication from the prying eyes of an eavesdropper. Yet, with the advent of modern communications new cryptographic challenges arose: we would like to enable two parties, Alice and Bob, to solve joint problems even if they do not trust each other. Examples of such tasks include secure auctions or the problem of secure identification such as that of a customer to an ATM. Although protocols for general two-party cryptographic problems may be very involved, it is known that they can in principle be built from basic cryptographic building blocks known as oblivious transfer [1] and bit commitment. The task of bit commitment is thereby particularly simple and has received considerable attention in quantum information. Intuitively, a bit commitment protocol consists of two phases. In the commit phase, Alice provides Bob with some form of evidence that she has chosen a particular bit C ∈ {0,1}. Later on in the open phase, Alice reveals C to Bob. A bit commitment protocol is secure if Bob cannot gain any information about C before the open phase, and yet, Alice cannot convince Bob to accept an opening of any bit . Unfortunately, it has been shown that even using quantum communication none of these tasks can be implemented securely [2] , [3] , [4] , [5] , [6] . Note that in quantum key distribution (QKD), Alice and Bob trust each other and want to defend themselves against an outsider Eve. This allows Alice and Bob to perform checks on what Eve may have done, ruling out many forms of attacks. This is in sharp contrast to two-party cryptography where there is no Eve, and Alice and Bob do not trust each other. Intuitively, it is this lack of trust that makes the problem considerably harder. Nevertheless, because two-party protocols form a central part of modern cryptography, one is willing to make assumptions on how powerful an attacker can be to implement them securely. Here we consider physical assumptions that enable us to solve such tasks. In particular, can the sole assumption of a limited storage device lead to security? [7] This is indeed the case and it was shown that security can be obtained if the attacker’s classical storage is limited [7] , [8] . Yet, apart from the fact that classical storage is cheap and plentiful, assuming a limited classical storage has one rather crucial caveat: if the honest players need to store N classical bits to execute the protocol in the first place, then any classical protocol can be broken if the attacker can store more than roughly N 2 bits [9] . Motivated by this unsatisfactory gap, it was thus suggested to assume that the attacker’s quantum storage was bounded [10] , [11] , [12] , [13] , [14] , or more generally, noisy [15] , [16] , [17] . The central assumption of the noisy-storage model is that during waiting times Δ t introduced in the protocol, the attacker can only keep quantum information in his quantum storage device . The exact amount of noise can depend on the waiting time. Otherwise, the attacker may be all powerful. In particular, he can store an unlimited amount of classical information, and perform any computation instantaneously without errors. Note that the latter implies that the attacker could encode his quantum information into an arbitrarily complicated error-correcting code, to protect it from noise in his storage device . The assumption that storing a large amount of quantum information is difficult, is indeed realistic today, as constructing large-scale quantum memories that can store arbitrary information successfully in the first attempt has proved rather challenging. We emphasize that this model is not in contrast with our ability to build quantum repeaters, where it is sufficient for the latter to store quantum states while making many attempts. A review on quantum memories can be found in Lvovsky et al. , [18] and numerous recent work can also be found in Usmani et al. , [19] Bonarota et al. , [20] and Dai et al. [21] While noting that perpetual advances in building quantum memories fundamentally affect the feasibility of all protocols in the noisy-storage model, we will explain below that given any upper bound on the size and noisiness of a future quantum storage device, security is in fact possible—we merely need to send more qubits during the protocol. In this work, we have implemented a bit commitment protocol that is secure under the noisy-storage assumption. We provide a general security analysis of our protocol for a range of possible experimental parameters. The parameters of our particular experiment are shown to lie within the secure region. The storage assumption in our work is such that a cheating party cannot store ≳ 900 qubits, which is a reasonable physical constraint given modern day technology of storing quantum information. The noisy-storage model To state our result, let us first explain what we mean by a quantum storage device, and how an assumption regarding these devices translates to security conditions in the noisy-storage model. A more detailed introduction to the model can be found in König et al. [17] Of particular interest to us are storage devices consisting of S ‘memory cells’, each of which may experience some noise itself. Mathematically, this means that the storage device is a quantum channel (a completely positive trace preserving map) of the form , where is a noisy channel acting on each memory cell, mapping input states to some noisy output states. For example, a noise-free storage device consisting of S qubits (that is, d =2) corresponding to the special case of bounded storage [12] is given by , where is the identity channel with one qubit input and one qubit output. Another example is a memory consisting of S qubits, each of which experiences depolarizing noise according to the channel . The larger r is, the less noise is present. Yet, another example is the erasure channel, which models losses in the storage device. It is indeed intuitive that security should be related to ‘how much’ information the attacker can squeeze through his storage device. That is, one expects a relation between security and the capacity of to carry quantum information. Indeed, it was shown that security can be linked to the classical capacity [17] , the entanglement cost [22] , and finally the quantum capacity [23] of the adversary’s storage device . When evaluating security, we start with a basic assumption on the maximum size and the minimum amount of noise in an adversary’s storage device. Such an assumption can for example be derived by a cautious estimate based on quantum memories that are available today. Note that these assumptions are for memories that can store arbitrary states on first attempt. Such memories presently exist for a handful of qubits. Given such an estimate, we then determine the number of qubits we need to transmit during the protocol to effectively overflow the adversary’s memory device and achieve security. Protocol and its security We consider the bit commitment protocol from König et al. [17] with several modifications to make it suitable for an experimental implementation with time-correlated photon pairs. 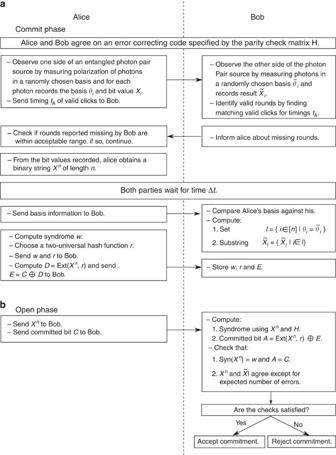Figure 1: Flowchart of the bit commitment protocol. This protocol allows Alice to commit a single bitC∈{0,1}. Alice holds the source that creates the entangled photon pairs. The function Syn maps the binary stringXnto its syndrome as specified by the error-correcting code. The function Ext: {0,1}n→{0,1} is a hash function indexed byr, performing privacy amplification. We refer to theSupplementary Methodsfor a more detailed statement of the protocol including details on the acceptable range of losses and errors. Note that the protocol itself does not require any quantum storage to execute. Figure 1 provides a simplified version of this modified protocol without explicit parameters—the explicit version can be found in the Supplementary Methods . In the Supplementary Methods , we also provide a general analysis that can be used for any experimental setup (details on our particular experiment are also provided in the same section). Figure 1: Flowchart of the bit commitment protocol. This protocol allows Alice to commit a single bit C ∈ {0,1}. Alice holds the source that creates the entangled photon pairs. The function Syn maps the binary string X n to its syndrome as specified by the error-correcting code. The function Ext: {0,1} n →{0,1} is a hash function indexed by r , performing privacy amplification. We refer to the Supplementary Methods for a more detailed statement of the protocol including details on the acceptable range of losses and errors. Note that the protocol itself does not require any quantum storage to execute. Full size image To understand the security constraints, we first need to establish some basic terminology. In our experiment, Alice holds the source, and both Alice and Bob have four detectors, each one corresponding to one of the four BB84 states [10] . If Alice or Bob observes a click of exactly one of their detectors (symmetrized with the procedure outlined in Supplementary Methods ), we refer to it as a valid click. Cases where more than one detector clicks at the same instant on the same side are ignored. A round is defined by a valid click of Alice’s detectors. A valid round is where both parties Alice and Bob registered a valid click in a corresponding time window, that is, where a photon pair has been identified. First, to deal with losses in the channel we introduce a new step in which Bob reports a loss if he did not observe a valid click. Second, to deal with bit flip errors on the channel, we employ a different class of error-correcting codes, namely a random code. Usage of random codes is sufficient for this protocol, as decoding is not required for honest parties. The main challenge is then to link the properties of random codes to the protocol security. Before we can argue about the correctness and security of the proposed protocol, let us introduce four crucial figures of interest that need to be determined in any experimental setup. The first two are the probabilities and , that none or just a single photon was sent to Bob, respectively, conditioned on the event that Alice observed a round. The third is the probability that honest Bob registers a round as missing, that is Bob does not observe a valid click when Alice does. Again, this probability is conditioned on the event that Alice observed a round. Note that by no-signalling, Alice’s choice of better (or worse) detectors should not influence the probability of Bob observing a round. Finally, we will need the probability p err of a bit flip error, that is the probability that Bob outputs the wrong bit even though he measured in the correct basis. Naturally, as Alice and Bob do not trust each other, they cannot rely on each other to perform said estimation process. Note, however, that the scenario of interest in two-party cryptography is that the honest parties essentially purchase off the shelf devices with standard properties, for which either of them could perform said estimate. It is only the dishonest parties who may be using alternate equipment. Another way to look at this is to say that there exists some set of parameters (that is, maximum losses, maxmium amount of noise on the channel, and so on) such that an honest party has to conform to these requirements when executing the protocol. Let us now sketch why the proposed protocol remains correct and secure even in the presence of experimental errors. A detailed analysis is provided in the Supplementary Methods . In our analysis, we take the storage device , as well as a fixed overall security error ɛ as given. Let M be the number of rounds Alice registers during the execution of the protocol. Let n be the number of valid rounds. In the description of theoretical parameters found in the Supplementary Methods , it is shown that M and n are directly related to each other, given some fixed experimental parameters. In particular, n is a function of M and We can now ask, how large does M (or equivalently n ) need to be to achieve security. If n is very small, for example if n ∼ 100, it is relatively easy to break the protocol, as a cheating party might be able to store enough qubits. Also many terms from our finite n analysis reach convergence only for sufficiently large n . As these terms depend on experimental parameters, security can be achieved for a larger range of experimental parameters if n is large. By fixing the assumption on quantum storage size, experimental parameters and security error values, our analysis allows us to determine a value of n where security is achievable. Correctness First of all, we must show that if Alice and Bob are both honest, then Bob will accept Alice’s honest opening of the bit C . Note that the only way that honest Bob will reject Alice’s opening is when too many errors occur on the channel, and hence part 2 of Bob’s final check (see Fig. 1 ) will fail. A standard Chernoff style bound using the Hoeffding inequality [24] shows the probability of this event is small, that is, the deviation from the expected number of p err n errors is not too large. Security against Alice Second, we must show that if Bob is honest, then Alice cannot get him to accept an opening of a bit . In our protocol, Alice is allowed to be all powerful, and is not restricted by any storage assumptions. If she is dishonest, we furthermore assume that she can even have perfect devices and can eliminate all errors and losses on the channel. The first part of our analysis, that is, the analysis of the steps before the syndrome is sent is thereby identical to Wehner et al. [25] (see Fig. 1 ). More precisely, it is shown that up to this step in the protocol, a string X n ∈ {0,1} n is generated such that Bob knows the bits for a randomly chosen subset , where corresponds to the entries of the string X n indexed by the positions in . If Alice is dishonest, we want to be sure at this stage that she cannot learn , that is, she cannot learn which bits of X n are known to Bob. In the original protocol without experimental imperfections [17] this was trivially guaranteed because Bob never sent any information to Alice. In this practical protocol, however, Bob does send some information to Bob, namely which rounds are valid for him, that is, when he saw a click. In Wehner et al. [25] it was simply assumed that the probability of Bob observing a loss is the same for all detectors, and hence in particular also independent of Bob’s basis choice. This is generally never the case in practise. However, by symmetrizing the losses as outlined in the Supplementary Methods , one can ensure that the losses become the same for all detectors. In essence, this procedure probabilistically adds additional losses to the better detectors such that in the end all detectors are as lossy as the worst one. As Bob’s losses are then independent of his basis choice, that is, the detectors, this is means that Alice cannot gain any information about when Bob reports some rounds as being lost. The second part of the protocol and its analysis uses the string X n and Bob’s partial knowledge to bind Alice to her commitment. First, we have that properties of the error-correcting code ensure that if the syndrome of the string (Syn( X n ) in Fig. 1 ) matches and Alice passes the first test, then she must flip many bits in the string to change her mind. In the original protocol of König et al. [17] sending Bob the syndrome of X n ensured that she must change at least bits of X n where d is the distance of the error-correcting code, such that Bob will accept the syndrome to be consistent. However, as Alice does not know which bits are known to Bob she will get caught with high probability. This is because of the fact that with probability 1−(1/2) d /2 Alice changed at least a bit known to Bob, and in the perfect case Bob aborts whenever a single bit is wrong. As we have to deal with experimental imperfections we cannot have that Bob aborts whenever a single bit is wrong, as bit flip errors on the channel likely lead errors even when Alice is honest. As such, the difference to the analysis of König et al. [17] is that Bob must accept some incorrect bits in part two of his final check (see Fig. 1 ). Our argument is nevertheless quite similar, but does require a careful tradeoff involving all experimental parameters between the distance of the code and the syndrome length (see below). We hence use a different error-correcting code as compared with König et al. [17] In particular, we use a random code, which has the property that with overwhelming probability its distance is large (that is it is hard for Alice to cheat), while nevertheless having a reasonably small syndrome length (see Supplementary Discussion ). The latter will be important in the security analysis below when Alice herself is honest. Security against Bob Finally, we must show that if Alice is honest, then Bob cannot learn any information about her bit C before the open phase. Again, dishonest Bob may have perfect devices and eliminate all errors and losses on the channel. His only restriction is that during the waiting time Δ t he can store quantum information only in the device . We first show that Bob’s information about the entire string X n is limited. We know from König et al. [17] that Bob’s min-entropy about the string X n before Alice sends the syndrome, given all his information including his quantum memory can be bounded by where is the maximum probability of transmitting Rn randomly chosen bits through the channel where R is called the rate. This rate is determined using a novel uncertainty relation that we prove for BB84 measurements, and all experimental parameters. The min-entropy itself can thereby be expressed as , where P guess ( X n |Bob) is the probability that Bob guesses the string X n , maximized over all measurements that he can perform on his system [26] . As Alice sends the syndrome to Bob, Bob gains some additional information which reduces his min-entropy. More precisely, it could shrink at most by the length of the syndrome, that is, Note that this is the reason why we asked for the error-correcting code to have a short syndrome length above. Finally, we show that knowing little about all of X n implies that Bob cannot learn anything about C itself. More precisely, when Alice chooses a random two universal hash function Ext ( X n , R ) and performs privacy amplification [27] , Bob knows essentially nothing about the output Ext ( X n , R )= D whenever his min-entropy about X n is sufficiently large. The bit D then acts as a key to encrypt the bit C using a one-time pad. As Bob cannot know D , he also cannot know C . Our analysis is thereby very similar to König et al. [17] , requiring only a very careful balance between the distance of the error-correcting code above, and the syndrome length. We provide a detailed analysis in the Supplementary Methods , where a general statement for arbitrary storage devices is included. Especially for the case of bounded storage , we can easily evaluate how large M needs to be, to achieve security against both Alice and Bob, when an error parameter ɛ is fixed. The total execution error of the protocol is obtained by adding up all sources of errors throughout the protocol analysis. The case where Alice and Bob are both dishonest is not of interest, because the aim of this protocol is to perform correctly while both players are honest, and protect the honest players from dishonest players. Experiment We have implemented a quantum protocol for bit commitment that is secure in the noisy-storage model. For this, n =250,000 valid rounds (see below) were used at a bit error rate of p err =4.1% (after symmetrization) to commit one bit with a security error of less than ɛ =2 × 10 −5 . Note that ɛ is the final correctness and security error for the execution of bit commitment in our experiment. This protocol is secure under the assumption that Bob’s storage size is no larger than 972 qubits, where each qubit undergoes a low depolarizing noise with a noise parameter r =0.9 (see Supplementary Methods ). We stress that our analysis is done for finite n , and all finite size effects and errors are accounted for. The ɛ includes the error in the choice of random code in the protocol, finite size effects that need to be bounded, smoothing parameters from an uncertainty relation, and so on. Our experimental implementation demonstrates for the first time that two-party protocols proposed in the bounded and noisy-storage models are well within today’s capabilities. We demonstrated, for the first time, that two-party protocols proposed in the bounded and noisy-storage models can be implemented today. We emphasize that whereas—similar to so many experiments in quantum information—our experiment is extremely similar to QKD the experimental parameter requirements and analysis is entirely different to QKD. Where there are many experiments carrying out QKD, there are only a handful of implementation results for two-party protocols [28] , [29] . Bit commitment is one of the most fundamental protocols in cryptography. For example, it is known that with bit commitment, coin tossing can be built. Also using additional quantum communication we can build oblivious transfer [30] , which in turn enables us to solve any two-party cryptographic problem [1] . In the Supplementary Methods , we provided a detailed analysis of our modified bit commitment protocol including a range of parameters for which security can be shown. Our analysis could be used to implement the same protocol using a different, technologically simpler setup, with potentially lower error rates or losses. Our analysis can also address the case of committing several bits at once. It would be interesting to see implementations of other protocols in the noisy-storage model. Finally, note that our analysis rests on a fundamental assumption made in in the analysis of all cryptographic protocols, namely that Alice does not have access to Bob’s lab and vice versa. In particular, this means that Alice cannot tamper with the random choices made by Bob, potentially forcing him to measure for example only in one basis, or by maniplating apparent detector losses [31] , [32] . Parameter ranges Our theoretical analysis shows security for a general range of parameters as illustrated in Figs 2 , 3 and 4 . A fully general theoretical statement can be found in the Supplementary Methods . These plots demonstrate that security is possible for a wide range of parameters, of which our particular implementation forms a special case. The plots are done for fixed values of n =250,000 and a total execution error of ɛ =3 × 10 −4 , unless otherwise indicated. Finally, Bob’s storage size is quantified by S , the number of qubits that Bob is able to store. The plots assume a memory of S qubits, where each qubit undergoes depolarizing noise with parameter r =0.9. 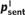Figure 2: Security region forversus. is set to be 0.765. Plots are for distinct values ofperr, whereas storage size is fixedS=2,500, and. For small values of(large amounts of losses), there exists a threshold onfor the protocol to be secure. This threshold increases withperr, and for extremely small storage rates, it gives a maximal tolerableperr∼0.046. Figure 2: Security region for versus . is set to be 0.765. Plots are for distinct values of p err , whereas storage size is fixed S =2,500, and . For small values of (large amounts of losses), there exists a threshold on for the protocol to be secure. This threshold increases with p err , and for extremely small storage rates, it gives a maximal tolerable p e rr ∼ 0.046. 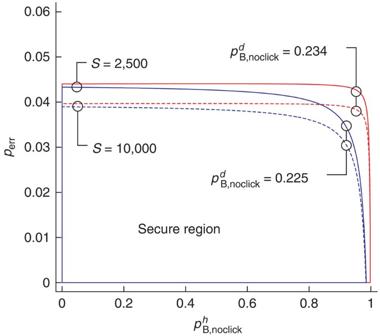Figure 3: Security region for some typical parameter ranges. andperrquantify the amount of erasures and errors in the protocol. For higher summation values of, the less multi-photons Bob gets, and erasures have less impact on the protocol security. This implies if the source is ideal, the protocol remains secure for large values of erasures. Dependences in the security region between erasures and errors also become more obvious whenis low. Furthermore, large assumptions onSdirectly decrease the amount of min-entropy, causing tolerableperrto drop consistently for all amounts of erasures. Full size image Figure 3: Security region for some typical parameter ranges. and p err quantify the amount of erasures and errors in the protocol. For higher summation values of , the less multi-photons Bob gets, and erasures have less impact on the protocol security. This implies if the source is ideal, the protocol remains secure for large values of erasures. Dependences in the security region between erasures and errors also become more obvious when is low. Furthermore, large assumptions on S directly decrease the amount of min-entropy, causing tolerable p err to drop consistently for all amounts of erasures. 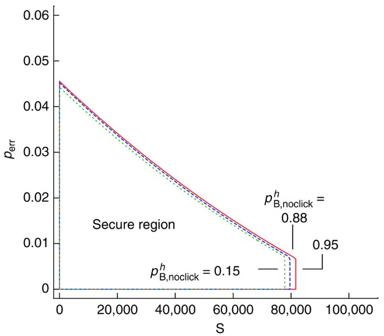Figure 4: Security region for different storage sizeSand error rateperr. Hereandare fixed. This plot shows a monotonic decreasing trend for tolerableperrwith respect to storage sizeS. The sharp cutoff forSvaries with, as with lower detection efficiency, dishonest Bob can report more missing rounds, hence the lower his storage size has to be for security to hold. Also, the plot shows security for mostly low values of storage rate. The result is non-optimal, as it has been shown22that security can be achieved with arbitrarily large storage sizes, if the depolarizing noise parameter. This is because we bound the smooth min-entropy of an adversarial Bob by the classical capacity of a quantum memory, whereas Bertaet al.22does so in terms of entanglement cost. As the latter is generally smaller than the former, this poses a better advantage for security, which is not shown in our analysis. Full size image Figure 4: Security region for different storage size S and error rate p err . Here and are fixed. This plot shows a monotonic decreasing trend for tolerable p err with respect to storage size S . The sharp cutoff for S varies with , as with lower detection efficiency, dishonest Bob can report more missing rounds, hence the lower his storage size has to be for security to hold. Also, the plot shows security for mostly low values of storage rate. The result is non-optimal, as it has been shown [22] that security can be achieved with arbitrarily large storage sizes, if the depolarizing noise parameter . This is because we bound the smooth min-entropy of an adversarial Bob by the classical capacity of a quantum memory, whereas Berta et al. [22] does so in terms of entanglement cost. As the latter is generally smaller than the former, this poses a better advantage for security, which is not shown in our analysis. Full size image Experimental implementation We implement this protocol with a series of entangled photons, with the polarization degree of freedom forming our qubits. This allows for reliable measurements in two complementary bases. Basis 1 corresponds to horizontal/vertical (HV) polarization, and basis 2 to ±45° linear polarization. The polarization-entangled photon pairs are prepared via spontaneous parametric down conversion (SPDC), collected into single-mode optical fibres, and guided to polarization analyser (PA) located with Alice and Bob (see Fig. 5 ). Each PA consists of a nonpolarizing beam splitter (BS) providing a random basis choice, followed by two polarizing beam splitters (PBS) and a pair of silicon avalanche photodiodes as single photon detectors in each of the BS outputs. A half-wave plate before one of the PBS rotates the polarization by 45°. This detection setup was used in a number of QKD demonstrations [33] , [34] , [35] . 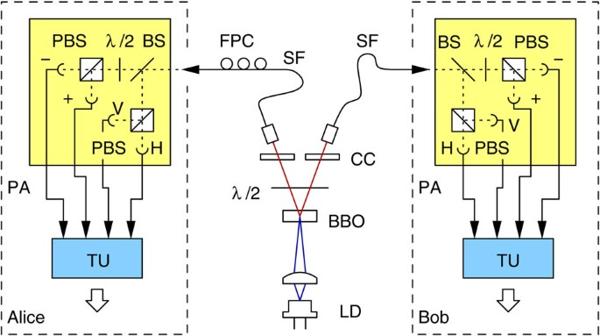Figure 5: Experimental setup. Polarization-entangled photon pairs are generated via non-collinear type-II SPDC of blue light from a laser diode (LD) in a barium–betaborate crystal (BBO), and distributed to PA at Alice and Bob via single-mode optical fibres (SF). The PA are based on a BS for a random measurement base choice, a half wave plate (λ/2) at one of the outputs, and PBS in front of single-photon counting silicon avalanche photodiodes. Detection events on both sides are timestamped (TU) and recorded for further processing. A polarization controller ensures that polarization anticorrelations are observed in all measurement bases. Figure 5: Experimental setup. Polarization-entangled photon pairs are generated via non-collinear type-II SPDC of blue light from a laser diode (LD) in a barium–betaborate crystal (BBO), and distributed to PA at Alice and Bob via single-mode optical fibres (SF). The PA are based on a BS for a random measurement base choice, a half wave plate ( λ /2) at one of the outputs, and PBS in front of single-photon counting silicon avalanche photodiodes. Detection events on both sides are timestamped (TU) and recorded for further processing. A polarization controller ensures that polarization anticorrelations are observed in all measurement bases. Full size image The SPDC source is similar to Ling et al., [35] with a continuous wave-free running laser diode (398 nm, 10 mW) pumping a 2 mm-thick Barium-betaborate crystal cut for type-II non-collinear parametric down conversion and the usual walkoff compensation to obtain polarization-entangled photon pairs [36] . We collect photon pairs into single mode optical fibres such that we observe an average pair rate r p =2,997±82 s −1 . Such a source generates photon pairs in a stochastic manner, but with a strong correlation in time. Therefore, valid clicks are timestamped on both sides first. In a classical communication step, detection times t A , t B are compared, and valid rounds are identified if valid clicks fall into a coincidence time window of τ c =3 ns, that is, | t A − t B |≤ τ c /2, similar to Marcikic et al. [34] with the code in Kurtsiefer [37] . The visibility of the polarization correlations in the singlet state are 97.7±0.6% and 94.7±0.9% in the HV and 45° linear basis. Individual detection rates on both sides are r A =23,758±221 s −1 and r B =22,227±247 s −1 on Alice and Bob’s side, respectively. In an initial alignment step, the fibre polarization controller was adjusted such that we see polarization correlations corresponding to a singlet state with a quantum bit error ratio of about p err =4.1%. The quantum bit error ratio is not to be confused with the failure probability of bit commitment protocol. Calculations of the latter are explicitly stated in the Supplementary Methods . As reported in the summarizing paragraph of our introduction, this quantity is much smaller than the former. For carrying out a successful bit commitment, we need to determine the parameters , , and . Depending on these probabilities and the desired error parameter ɛ , we choose a particular error-correcting code and number of rounds M needed for a successful bit commitment. To estimate these probabilities out of the experimental parameters of our source/detector combination, we model our setup by a lossless SPDC source emitting only photon pairs at a rate r s , and assign all imperfections (losses, limited detection efficiency and background events) to the detectors at Alice and Bob. As the coherence time of the photons in our case is much shorter than the coincidence detection time window τ c , the distribution of photon pairs in time can be well described by a Poisson process, which allows an assessment of multiphoton events. A detailed derivation of bounds for the probabilities is given in the Supplementary Methods , we just summarize the results necessary for evaluating the security of the protocol: Owing to small differences in the detection efficiency of the avalanche photodiodes and imperfections in polarization components in the actual experiment, there is an asymmetry in the probability of detecting each bit in each basis. Furthermore, the beam splitter for the random measurement basis choice are not completely balanced. A summary of these imperfections over a number of bit commitment runs is shown in Fig. 6 . This can be corrected for by discarding rounds until the probabilities for both bits are equal. Discarded bits can be modelled as losses without affecting the security of the protocol. A detailed analysis of this can be found in the Supplementary Methods . 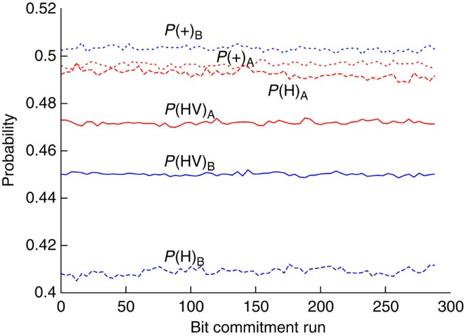Figure 6: Bias in measurements. Solid lines indicate the probabilitiesP(HV) of a HV basis choice for both Alice and Bob for data sets of 250,000 events each. Dashed lines indicate the probabilityP(H) of a H in the HV measurement basis, the dotted lines the probabilityP(+) of a +45° detection in a ±45° measurement basis. These asymmetries arise form optical component imperfections and are corrected in a symmetrization step. Figure 6: Bias in measurements. Solid lines indicate the probabilities P (HV) of a HV basis choice for both Alice and Bob for data sets of 250,000 events each. Dashed lines indicate the probability P (H) of a H in the HV measurement basis, the dotted lines the probability P (+) of a +45° detection in a ±45° measurement basis. These asymmetries arise form optical component imperfections and are corrected in a symmetrization step. Full size image How to cite this article: Ng, N.H.Y. et al. Experimental implementation of bit commitment in the noisy-storage model. Nat. Commun. 3:1326 doi: 10.1038/ncomms2268 (2012).